ThePHgene determines fruit acidity and contributes to the evolution of sweet melons Taste has been the subject of human selection in the evolution of agricultural crops, and acidity is one of the three major components of fleshy fruit taste, together with sugars and volatile flavour compounds. We identify a family of plant-specific genes with a major effect on fruit acidity by map-based cloning of C. melo PH gene ( CmPH ) from melon, Cucumis melo taking advantage of the novel natural genetic variation for both high and low fruit acidity in this species. Functional silencing of orthologous PH genes in two distantly related plant families, cucumber and tomato, produced low-acid, bland tasting fruit, showing that PH genes control fruit acidity across plant families. A four amino-acid duplication in CmPH distinguishes between primitive acidic varieties and modern dessert melons. This fortuitous mutation served as a preadaptive antecedent to the development of sweet melon cultigens in Central Asia over 1,000 years ago. Acidity is a major determinant of the taste and quality of most fruits, in combination with sugars and flavour volatiles [1] , [2] but the molecular–genetic control of plant acid levels has only been partially deciphered. Most edible fruits have acidic pH values in the range of 3–5. While genetic variation for fruit acidity has been identified in many fruit crops [3] , [4] , [5] , [6] , genes responsible have not yet been conclusively identified, even in major fruit crops such as grape, citrus, tomato, peach and apple, which have attracted extensive genomic, biochemical and physiological research attention [7] . A number of pH-associated genes have been characterized in flowers, due to the petal pigmentation phenotypes caused by the effect of pH on the spectra of flavonoids [8] , [9] , [10] , [11] . The cultivated sweet dessert melons, Cucumis melo L., are quite unique among fleshy fruit in that they have unusually low levels of acidity, with pH values in the near neutral range. This is in sharp contrast to the more primitive members of the species whose fruit are acidic when mature [12] , [13] , [14] , [15] . The genetic trait of sourness, or acidity, of melon fruit flesh is conferred by a single dominant locus termed So ( Sour ) or PH [14] , [15] , [16] . As all sweet melon accessions are non-acidic, they are homozygous for the recessive mutant, ph/ph . Therefore, the PH gene is intriguing, not only for understanding fruit physiology, but also for clarifying the sequence of molecular events contributing to crop species diversification. In this study, we identify a gene family encoding membrane proteins responsible for acidity in fruit, using a map-based cloning strategy based on the novel natural genetic variability for fruit acidity in melon. Orthologues are expressed in numerous species of fruit, and we show functionality of the gene in distantly related members of the plant family. The results presented here identify a plant-specific gene family responsible for the important trait of fruit acidity and reveal the fateful molecular evolutionary event that eventually led to the popularity and expansion of C. melo dessert melons around the globe. The identification of the PH gene The PH locus in melon was initially mapped to an ~2 cM region on the distal portion of chromosome 8 (ref. 15 ). An extensive mapping colocalization screen of the PH QTL with nearly 60 candidate genes, comprising those encoding fruit organic acid metabolism and the major H + transporters, did not support any of these as the PH gene [3] . We identified the PH gene using a map-based cloning strategy ( Fig. 1a and Supplementary Fig. 1 ) that involved two individual intraspecific segregating populations: an RIL (recombinant inbred lines) population derived from a cross of the high-pH muskmelon (Reticulatus group) ‘Dulce’ and the low-pH Indian phut snapmelon (Momordica group) PI414723 (ref. 15 ), and a near-isogenic pair of melon lines segregating for the pH trait ( Fig. 2a–c ), which were produced by crossing the high-pH cantaloupe (Cantalupensis group) ‘Noy Yizre‘el’ and the low-pH snake melon (Flexuosus group) ‘Faqqous’ [16] . 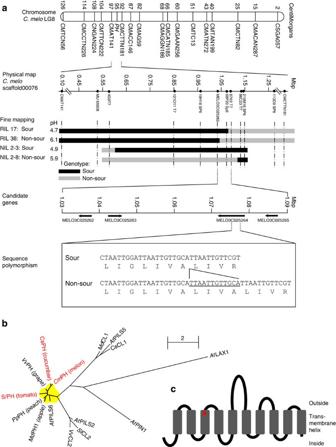Figure 1: Map-based cloning and phylogenetic position of theCmPHgene. (a) Top to bottom: the combined marker map (11) showingC. melolinkage group 8 with representative markers; the physical map (15) displaying a ~1 Mbp segment between two SSR markers harbouring thePHlocus; schematic genotypic representation of the key recombinant lines used to limit thePHlocus position (sour genotypes are indicated by black bars and non-sour genotypes by grey bars); candidate genes encoded by the ~50 Kb segment (gene accession numbers are fromwww.melonomics.net); sequence comparison of MELO3025264 from the sour and non-sour genotypes indicated a 12-bp duplication leading to four amino-acid duplications in the translated protein in the non-sour genotype. A more detailed map-cloning presentation, including a synteny map with cucumber is presented inSupplementary Fig. 1. (b) A radial, unrooted phylogenetic tree demonstrating the relationship (maximum likelihood) between PH proteins and other related plant transporter proteins. The clade corresponding to thePHgenes is coloured. Genes for which function has been shown in this study are coloured red.At,Arabidopsis thaliana;Md,Malus domestica;Cm,Cucumis melo;Cs,Cucumis sativus;Vv,Vitis vinifera;Sl,Solanum lycopersicon;Pp,Prunus persica. Cl1 and Cl2 refer to the related clades shown inSupplementary Fig. 2. The accession numbers of the proteins used for the preparation of this tree are listed inSupplementary Table 1. (c) Predicted likely topology of theCmPHprotein, based on 17 modelling programs, as described inSupplementary Fig. 3andSupplementary Data 1. The QTL was narrowed to an ~50 kB region harbouring four open reading frames (ORFs), only one of which is expressed in melon fruit ( Supplementary Table 1 , melon unigene MU46248, www.icugi.org ; MELO3C025264, www.melonomics.net [17] ). Figure 1: Map-based cloning and phylogenetic position of the CmPH gene. ( a ) Top to bottom: the combined marker map ( 11 ) showing C. melo linkage group 8 with representative markers; the physical map ( 15 ) displaying a ~1 Mbp segment between two SSR markers harbouring the PH locus; schematic genotypic representation of the key recombinant lines used to limit the PH locus position (sour genotypes are indicated by black bars and non-sour genotypes by grey bars); candidate genes encoded by the ~50 Kb segment (gene accession numbers are from www.melonomics.net ); sequence comparison of MELO3025264 from the sour and non-sour genotypes indicated a 12-bp duplication leading to four amino-acid duplications in the translated protein in the non-sour genotype. A more detailed map-cloning presentation, including a synteny map with cucumber is presented in Supplementary Fig. 1 . ( b ) A radial, unrooted phylogenetic tree demonstrating the relationship (maximum likelihood) between PH proteins and other related plant transporter proteins. The clade corresponding to the PH genes is coloured. Genes for which function has been shown in this study are coloured red. At , Arabidopsis thaliana ; Md , Malus domestica ; Cm , Cucumis melo ; Cs , Cucumis sativus ; Vv , Vitis vinifera ; Sl , Solanum lycopersicon ; Pp , Prunus persica . Cl1 and Cl2 refer to the related clades shown in Supplementary Fig. 2 . The accession numbers of the proteins used for the preparation of this tree are listed in Supplementary Table 1 . ( c ) Predicted likely topology of the CmPH protein, based on 17 modelling programs, as described in Supplementary Fig. 3 and Supplementary Data 1 . 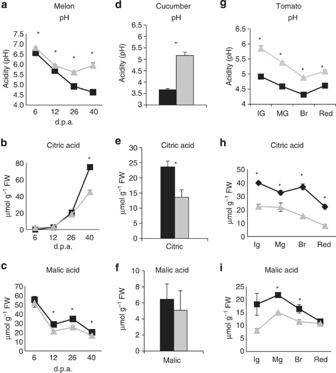Figure 2: Citrate, malate and pH levels in fruit with alteredPHexpression. (a–c) Near-isogenic melon genotypes through fruit development, (d–f) mature transgenic, silenced and non-silenced cucumber fruit and (g–i) transgenic, silenced and non-silenced tomato fruit through fruit development. Grey lines and bars represent the low-acid genotypes and black lines and bars represent the high-acid genotypes. FW, fresh weight; IG, immature green; MG, mature green; Br, breaker; R, red; d.p.a., days post anthesis. Additional metabolites are presented inSupplementary Figs 4 and 5. Error bars are s.e.m. of three biological replicates. Asterisks indicate significant differences (P<0.05;n=3; for (d) and (g)n=2), as determined using Student’st-test. Full size image Figure 2: Citrate, malate and pH levels in fruit with altered PH expression. ( a – c ) Near-isogenic melon genotypes through fruit development, ( d – f ) mature transgenic, silenced and non-silenced cucumber fruit and ( g – i ) transgenic, silenced and non-silenced tomato fruit through fruit development. Grey lines and bars represent the low-acid genotypes and black lines and bars represent the high-acid genotypes. FW, fresh weight; IG, immature green; MG, mature green; Br, breaker; R, red; d.p.a., days post anthesis. Additional metabolites are presented in Supplementary Figs 4 and 5 . Error bars are s.e.m. of three biological replicates. Asterisks indicate significant differences ( P <0.05; n= 3; for ( d ) and ( g ) n =2), as determined using Student’s t -test. Full size image In order to verify the identity of the PH gene, and in the absence of a genetic transformation system for the primitive acidic melons, stable silencing transformation was performed in the sister species Cucumis sativus (cucumber), which expresses a nearly identical (97% amino-acid sequence identity) syntenic orthologous gene (Csa4g337340, Supplementary Fig. 1 ). Ripe cucumber fruit are sour and characterized by acidic pH of ~4 (ref. 18 ), similar to the low-pH melons. Our results clearly show that silencing the PH gene had a major effect on fruit acidity, reducing the acid levels in developing cucumber fruit ( Fig. 2d–f ) and yielding a non-sour mature fruit, readily recognizable by its bland taste. BLAST and phylogenetic analyses based on sequence similarities with C. melo PH gene ( CmPH ) indicated a family of proteins that are conserved and expressed in nearly all of the fruit species examined ( Table 1 ), in addition to the Cucurbitaceae (melon, cucumber, watermelon). These taxa include representatives from all of the major families with edible, cultivated fruit, including Solanaceae (tomato), Rosaceae (apple), Viticeae (grape) and Rutaceae (citrus). These proteins form a distinct clade, sharing >60% sequence identity ( Fig. 1b , Supplementary Fig. 2 ). Table 1 Genetic expression profiles of the PH gene in reproductive tissues of various plant species. Full size table Proving function of the PH genes In order to prove the functional orthology of the genes from other plant families, we prepared stable RNA interference (RNAi) transgenics of the ortholog in tomato and the results confirmed that the tomato PH ortholog controls fruit acidity in that species, as well. Fruit juice of the silenced T 1 plants had nearly a full pH unit increase throughout development compared with the non-silenced plants, together with reduced citric and malic acid levels ( Fig. 2g–i ), and the silenced ripe fruit had a distinctly non-sour, bland taste, as compared with the normal tomato. The protein is annotated as a member of the pfam 03547 membrane transporter family, and modelling indicates the presence of 10 transmembrane domains ( Fig. 1c , Supplementary Fig. 3 , Supplementary Data 1 ). The closest functionally characterized members of this family are the PIN H + /auxin transporters and some of the PIN-like (PILs) proteins, but these share less than 30% identity with the PH proteins [19] , [20] (clades I and II in Fig. 1b and Supplementary Fig. S2 ). The Arabidopsis gene AtPILs6 belongs to the PH clade but studies of the PILs family did not uncover any function related to auxin transport for this particular PH ortholog [19] . Similarly, we did not observe any auxin-related phenotype in the silenced tomato lines, whether in early seedling development or plant vegetative or reproductive development, and the low-acid melon and cucumber lines also did not display any visual phenotypes characteristic of disruption of auxin homeostasis. The protein was localized to the endoplasmic reticulum in a number of expression systems, including transient expression via agro infiltration in melon fruit; leaves, stem and ovary of stably transformed tobacco plants; protoplasts and isolated vacuoles from stably transformed tobacco leaves; and transient expression in yeast ( Fig. 3 ). The observed ER localization is consistent with that of some other plant H + transporters, including the orthologous AtPILs6 protein [19] , [20] , [21] , [22] , although it is surprising considering that fruit acidity is presumed to be compartmentalized in the vacuole [7] . 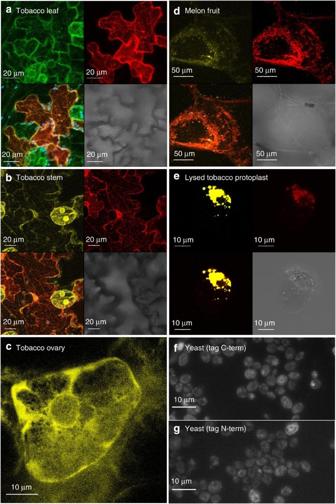Figure 3: Organellar localization of tomato PH protein. (a–e) YFP-PH or PH-GFP (yellow amino-terminal fluorescent tag or green carboxy-terminal fluorescent tag, respectively) expression in stable transgenic tobacco. (a) Tobacco leaf epidermal cells; (b) stem cells; (c) immature ovary; (d) transient YFP-PH and HDEL-RFP coexpression in young melon fruit. The micrograph of melon fruit is a three-dimensional reconstruction; (e) YFP-PH (yellow) in lysed tobacco protoplasts showing the fluorescence in the cytoplasmic components attached to the vacuole but not on the tonoplast membrane; (f) C-terminal fluorescent tag imaged in WT yeast cells (lens × 100). (g) N-terminal fluorescent tag imaged in WT yeast cells (lens × 100). In bothfandg, PH is targeted to the endoplasmic reticulum, as is evident from the double ring-like pattern visualized in the yeast. In composite figuresa,b,dande, PH with fluorescent tag is dyed in yellow or green (top left corner), transient HDEL-RFP expression in red (top right corner), the combined fluorescence in orange (bottom left corner) and clear field in grey (bottom right corner). Figure 3: Organellar localization of tomato PH protein. ( a – e ) YFP-PH or PH-GFP (yellow amino-terminal fluorescent tag or green carboxy-terminal fluorescent tag, respectively) expression in stable transgenic tobacco. ( a ) Tobacco leaf epidermal cells; ( b ) stem cells; ( c ) immature ovary; ( d ) transient YFP-PH and HDEL-RFP coexpression in young melon fruit. The micrograph of melon fruit is a three-dimensional reconstruction; ( e ) YFP-PH (yellow) in lysed tobacco protoplasts showing the fluorescence in the cytoplasmic components attached to the vacuole but not on the tonoplast membrane; ( f ) C-terminal fluorescent tag imaged in WT yeast cells (lens × 100). ( g ) N-terminal fluorescent tag imaged in WT yeast cells (lens × 100). In both f and g , PH is targeted to the endoplasmic reticulum, as is evident from the double ring-like pattern visualized in the yeast. In composite figures a , b , d and e , PH with fluorescent tag is dyed in yellow or green (top left corner), transient HDEL-RFP expression in red (top right corner), the combined fluorescence in orange (bottom left corner) and clear field in grey (bottom right corner). Full size image In an attempt to shed light on the function of the gene, we searched for metabolites that changed in a common and consistent manner between high- and low-acid fruits of all three species studied: melon, tomato and cucumber. We carried out a cross-species comparative metabolic profiling using non-targeted gas chromatography–mass spectrometry and liquid chromatography–mass spectrometry (LC–MS) metabolomic analyses and the only metabolites that behaved in a similar manner across all three species were, besides the major organic acids citrate and malate, surprisingly, the nucleosides adenosine and uridine ( Supplementary Figs 4 and 5 , Supplementary Data 2–5 ). In fruits of the low-acid line of melon, as well as the PH -silenced cucumber and tomato, the levels of organic acids were decreased while nucleoside levels were increased, as compared with the high-acid lines. We cannot claim at present whether organic acids or nucleosides are directly transported by the PH protein. The protein has little homology to any of the known organic acid or nucleoside transporters. Uptake and efflux experiments with organic acids or nucleosides in yeast did not indicate transport function with either ( Supplementary Fig. 6 ) and the gene did not complement either adenosine or uridine uptake mutants in yeast. Nevertheless, the PH protein, even in the absence of direct transporter activity, may indirectly play a role in nucleoside and organic acid homeostasis, either via modifications of a proton gradient or nucleoside and acid metabolism. Results of adenosine levels in yeast following adenosine feeding indicate that there seems to be an effect on adenosine homeostasis, irrespective of a direct transport role ( Supplementary Fig. 7 ). Recently, PH1 of petunia, a putative proton transporter, was shown to indirectly function in acidification by protein–protein interaction with the PH5 transporter, although it was incapable by itself of carrying out proton transport in heterologous expression systems [11] . Mutation of the PH gene led to low-acid sweet melons The ph/ph mutation that causes a low-acidity phenotype in melon is in the protein sequence and is not due to transcriptional or post-transcriptional changes. Comparative gene expression analysis did not indicate any transcriptional differences during fruit development and CmPH expression was similar in both sour and non-sour melon genotypes ( Supplementary Fig. 8 ). On the other hand, sequence comparison of the PH gene from the four parental genotypes of the melon mapping populations showed that the two non-sour melon genotypes (the muskmelon ‘Dulce’ and the cantaloupe ‘Noy Yizre‘el’) had identical four amino-acid duplications in the otherwise highly conserved third TMD ( Fig. 1a,c ). This duplication likely affects the structure of the transporter, by extending or shifting the third transmembrane domain to include the duplicated amino acids ( Supplementary Fig. 3 ). As the third TM is predicted to be longer than the others in the non-mutant protein (25 aa as compared with mostly 20-21 aa), any extension or shift is likely to adversely affect the functioning of the transporter. In order to explore the evolutionary history of the low-acid trait in melon and to substantiate the relationship between the mutant genotype and its phenotype, we surveyed 50 accessions of C. melo representing most of its cultivar groups and the broad genetic variability of the species ( Fig. 4a , Supplementary Data 6 ). Sweet melons comprise only some of the designated cultivar Groups of C. melo [12] , and include muskmelons (Reticulatus Group), cantaloupes (Cantalupensis Group), casabas (Inodorous Group), dry land sweet melons (Ameri Group) and Oriental sweet melons (Makuwa Group). These melons are consumed when fully ripe and sweet. When immature, they are bland, since sucrose only begins to accumulate in the fruits as they approach maturity. The fruits of other melon cultivar-groups, however, do not become sweet and instead become acidic and sour tasting upon ripening. Among these are the snake melons (Flexuosus Group) and chate melons (Adzhur Group), which are grown across much of northern Africa and southwestern, central and southern Asia and are consumed when immature, much like cucumbers, before they become acidic. Another important acidic, non-sweet group comprises the phut or snapmelons (Momordica group), which are widely grown in India. The acidity level and PH gene sequence of mature fruits of each accession were characterized and the results clearly show that the four amino-acid duplications are closely associated with the loss of fruit acidity throughout the species ( Fig. 4b ). Furthermore, sequence analysis shows that the 12-bp duplication is identical among all the non-acidic accessions, irrespective of cultivar-group ( Supplementary Fig. 9 ). 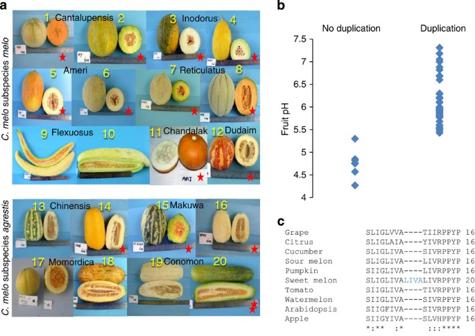Figure 4: Occurrence of the 12-bp duplication in theCmPHallele and the relation to fruit acidity. (a) Fruit phenotypes of representativeC. meloaccessions of the subsp.melo(top) and subsp.agrestis(bottom), indicating cultivar group relationships and the presence (red star) of the 12-bp duplication. The cultivars are described in detail inSupplementary Data 6. Accessions shown are (1) Védrantais, (2) Noy Yizre‘el, (3) Piel de Sapo, (4) Amarillo Oro, (5) Ananas Yoqne‘am, (6) Ananas En Dor, (7) Fordhook Gem, (8) Hale’s Best Jumbo, (9) Doya, (10) Armenian Yard Long, (11) Arka Jeet, (12) Dudaim, (13) PI 157071, (14) Ohgon, (15) PI 163375, (16) Batley’s Hermaphrodite, (17) MR1, (18) PI 414723, (19) Tokyo Giant, (20) Black Skin. (b) Correlation between the duplication genotype and fruit acidity amongC. melolines. Each data point indicates one of the 50 accessions described inSupplementary Data 6andSupplementary Fig. 7. (c) Alignment of the third TMD amino-acid sequence ofPHgene orthologs. The gene accessions presented in the alignment are described inSupplementary Table 2. Figure 4: Occurrence of the 12-bp duplication in the CmPH allele and the relation to fruit acidity. ( a ) Fruit phenotypes of representative C. melo accessions of the subsp. melo (top) and subsp. agrestis (bottom), indicating cultivar group relationships and the presence (red star) of the 12-bp duplication. The cultivars are described in detail in Supplementary Data 6 . Accessions shown are (1) Védrantais, (2) Noy Yizre‘el, (3) Piel de Sapo, (4) Amarillo Oro, (5) Ananas Yoqne‘am, (6) Ananas En Dor, (7) Fordhook Gem, (8) Hale’s Best Jumbo, (9) Doya, (10) Armenian Yard Long, (11) Arka Jeet, (12) Dudaim, (13) PI 157071, (14) Ohgon, (15) PI 163375, (16) Batley’s Hermaphrodite, (17) MR1, (18) PI 414723, (19) Tokyo Giant, (20) Black Skin. ( b ) Correlation between the duplication genotype and fruit acidity among C. melo lines. Each data point indicates one of the 50 accessions described in Supplementary Data 6 and Supplementary Fig. 7 . ( c ) Alignment of the third TMD amino-acid sequence of PH gene orthologs. The gene accessions presented in the alignment are described in Supplementary Table 2 . Full size image The acidic genotype is most likely the wild type, ancestral form. Orthologues of the PH gene in the Cucurbitaceae , including C. sativus L., Citrullus lanatus (Thunb.) Matsum. and Nakai and Cucurbita pepo L., and orthologues in other plant families ( Fig. 4c ) lack the four amino-acid duplications, which is found only in the non-acidic accessions of the melon species. The identical duplication/mutation in all of the non-acidic genotypes, irrespective of cultivar group, would seem to indicate a single molecular evolutionary event. Surprisingly, mutant non-sour genotypes are found not only among the muskmelons, cantaloupes and casabas of C. melo subspecies melo , but also among the more distantly related Oriental sweet melons of C. melo subspecies agrestis ( Fig. 4a ). A similar anomalous distribution in the widely divergent accessions of melon has been reported for a mutant sex type, andromonoecious [23] . In light of these results, it is interesting to speculate about the possible origin of sweet melon cultivation. C. melo is of Asian origin [24] and considerable diversity of wild melons has been described in India [25] . Apparently, melon types were domesticated thousands of years ago and dispersed widely by early historical times. Elongate melons of the acidic Adzhur and Flexuosus groups, as depicted in ancient Egyptian wall paintings, were the most widely mentioned and illustrated cucurbit in Mediterranean antiquity [26] . Among the domesticated Cucurbitaceae , fruit elongation is strongly associated with the culinary use of immature fruits [27] and many elongated varieties of melon are grown for their young, immature fruits, which are consumed fresh or pickled, like cucumbers. These immature fruits are not yet acidic, as the acidity accumulates only during the later stages of fruit development [16] . Round melons, used when ripe, were considered by Pliny (1st century CE) to be a new introduction [28] . However, they were not highly esteemed, as the praise so often associated with the organoleptic qualities of sweet melons is lacking. These newly introduced, round melons may have differed from their predecessors by not being sour, a characteristic which would have derived from a recessive mutation at the PH locus, resulting in ph/ph palatable, non-sour, though bland mature fruits. In fact, modern landraces of the Adana Group, named after a city adjacent to an intensively cultivated plain in southern Turkey, yield melons with mealy, non-sour, insipid to slightly sweet flesh that are consumed when mature [12] , [13] . Truly sweet melons originated in Khorasan, Central Asia by early medieval times and were subsequently dispersed westward [27] . Accordingly, the loss of fruit acidity in C. melo due to the 12-bp duplication is an example of a preadaptive molecular evolutionary event that has contributed to crop diversification, rather than to crop domestication in the strict sense. Purugannan and Fuller [29] pointed out that while most domestication genes (such as seed shattering [30] , [31] ) encode transcriptional activators, diversification genes (such as rice stickiness [32] ) are more likely to encode proteins with metabolic functions, such as enzymes or transporters. The absence of the combination of high-sugar and high-acid levels among existing sweet melon cultivars is not due to physiological constraints of combining the two taste components and, in fact, this combination has been attained in recent breeding programs [16] , [33] . Rather, it indicates that sweet dessert melons were selected from a limited pool of non-acidic, ph/ph mutant genotypes in Central Asia over 1,000 years ago. This may explain the narrow genetic base of sweet melon germplasm, which has necessitated the introgression of disease resistance from primitive acidic melons [25] and, simultaneously, offers new opportunities for the development of recombinant melons possessing unique combinations of quality attributes. We identified the PH gene in melon, exploiting a fortuitous mutation with a major impact on fruit acidity. Other plant families express orthologous genes, especially in their fruits. We have also shown that the cucumber and tomato orthologues of this gene do indeed play a role in controlling fruit pH. These results reveal the first family of plant-specific genes controlling fruit acidity and will likely impact on the manipulation of the important trait of acidity in fruits. Further investigations of the mode of action of the membrane transporter might reveal how cellular pH, in general, and fruit acidity in particular, are regulated. PH accession codes Sequence data used in this article is accessible at International Cucurbit Genome Initiative (ICuGI; www.icugi.org ), Spanish melon genome Consortium ( http://www.melogene.net ) or GenBank/NCBI ( http://www.ncbi.nlm.nih.gov ) under the accession numbers KJ704798 (‘PI414723’) and KJ704799 (`Dulce'). Plant material and growth conditions Parental lines . True-breeding melon ( C. melo) lines (minimum F 6 lines of C. melo Reticulatus Group `Dulce' and Momordica Group ‘PI414723’) were grown using standard cultural practices. Flowers were tagged at anthesis and a maximum of two fruits were allowed to develop per plant. Fruits were sampled at 10, 20, 30 and 40 days after anthesis. Melon accessions . Ripe fruits of the 50 accessions from the germplasm collection of melons maintained at the A.R.O. Newe Ya‘ar Center were sampled for TSS and pH ( Supplementary Data 6 ). Melon RILs (recombinant inbred lines) . A recombinant inbred melon population was developed from a cross between ‘PI414723’-S 5 ( C. melo Momordica Group) and ‘Dulce’ ( C. melo Reticulatus group) [15] . F 2 individuals ( n =112) originating from two F 1 plants were propagated by single-seed descent to create the population, which consisted of 99 F 6 -, F 7 - and F 8 -generation RI lines. Melon NILs (near-isogenic lines) . NILs were developed from the crossing of the sour and non-sour phenotypes, A6-Bc1S8 and F63-Bc3S7, respectively, initially developed from a cross between the non-sour ‘Noy Yizre‘el’ ( C. melo Cantalupensis group) and the sour 'Faqqous' ( C. melo Flexuosus group) [16] . Heterozygous individuals from the cross of A6-Bc1S8 and F63-Bc3S7 were self-pollinated and heterozygous selections were subsequently selfed through the F 7 , resulting in four homogenous F 8 lines, two of which had sour fruits, 236-1-3-2-3 and 236-1-3-3-1, and two of which had non-sour fruits, 236-1-3-2-8 and 236-1-3-3-2. Other plants were grown as follows: Tomatoes: Tomato ( Solanum lycopersicum ) plants were grown in the greenhouse under standard conditions, as previously described [34] . Var. ‘MP-1’ was used for the preparation of transgenic plants [35] . Cucumbers: Cucumber ( C. sativus ) plants were grown in a heated greenhouse using standard conditions. The variety ‘Ilan’ (Zera‘im Gedera, Gedera, Israel; http://www.zeraim.com ) was used as the line for transgenesis [36] and the ‘Derby’ (Hishtil, Ashqelon, Israel, http://www.hishtil.com ) line was grown as pollinator. Tobacco: Tobacco ( Nicotiana tabacum ) plants (var. ‘Samsun NN’) were grown in conditions described in ref. 37 . Fine mapping The physical mapping of the PH gene was completed using a set of melon BAC library filters (CM_MBa, Clemson University Genomic Institute, Clemson, South Carolina, USA, http://www.genome.clemson.edu ) screened with radioactive probes, as described previously [38] . In this manner, a contig of 16 BACS was developed, between the markers CMAT141 and MU57438, which was identified as being linked to the pH trait by a bulked segregant analysis strategy based on hybridization to a melon microarray [39] , [40] and served as a marker proximal to CMCTTN181 ( Supplementary Fig. 1 ). The contig gap between BAC 219J14 and 14B14 was bridged by the cucumber genomic scaffold based on melon homologues of Csa4G335230 and the melon genomic sequence of the flanking BAC ends. The completed contig was confirmed by the melon genome ( http://www.melogene.net ) that was generously opened to us prepublication [17] . Thirteen recombinants were observed between the two markers ( Supplementary Fig. 1 ). The analysis of the fruit pH phenotype of the recombinants allowed for the narrowing of the melon region harbouring the PH gene to ~50 kb interval. Comparison of the syntenous published cucumber and melon genomes led to the identification of four melon ORFs (MELO3C025262—MELO3C025265) in the region, described in Supplementary Table 1 . Molecular biology, Cloning and DNA constructs Primers: Primers used in this study are listed in Supplementary Table 2 . Full-length melon PH gene: The full-length sequence of the CmPH was amplified via PCR from cDNA extracted from ‘PI414723’ (1,242 bp) or ‘Dulce’ (1,254 bp) melon fruit using gene-specific primers ( Supplementary Table 2 ). Full-length tomato PH gene: The full-length S. lycopersicum PH ( SlPH ) ortholog (1,247 bp; Solyc10g074790.1.1) was identified by NCBI nucleic acid and translated protein databases and BLAST software and cloned via gene-specific primers ( Supplementary Table 2 ). RNAi constructs: Constructs for the silencing of the cucumber and tomato PH genes were developed using the RNAi pHannibal vector [41] . Primers for the construction of the melon and tomato silencing vectors (RNAi– CmPH and RNAi– SlPH , respectively) are listed in Supplementary Table 2 . The PCR products with their pHannibal flanking elements (CaMV 35-S and OCS terminator) were inserted into pGreen 0029 (ref. 41 ) resulting in the melon (pGreen–RNAi– CmPH ) and tomato (pGreen–RNAi– SlPH ) silencing vector. YFP-SlPH constructs: The fluorescent YFP marker for transient/stable expression of SlPH was based on the pSAT6-EYFP-C1 vector [42] (accession no. AY818380). The cloned full-length tomato PH gene served as template for a PCR using the primers YFP-SlPH ( Supplementary Table 2 ). This product was inserted downstream to the YFP gene in the pSAT6-EYFP-C1, and subsequently transferred with its flanking elements (2 × 35-S 5′ UTR and EYFP ) into the plant expression vector pGreen 0029 resulting in pGreen- YFP - SlPH , and into the yeast expression vector pESC-URA (Agilent Technologies, www.genomics.agilent.com ) resulting in pESC- YFP - SlPH . SlPH-GFP (green fluorescent protein) constructs: The fluorescent GFP marker for transient expression was based on the pART7-eGFP vector described by Avisar et al . [43] The full-length tomato PH gene served as template for a PCR using the SIPH - GFP primers ( Supplementary Table 2 ). This product was inserted upstream to the GFP gene in pART7-eGFP, and transferred, with its newly flanking elements (35-S, GFP and OCS 3′) into pGreen 0029, ensuing pGreen- SlPH-GFP , and into pESC-URA resulting in pESC- SlPH-GFP . Entry and Destination Gateway Vector Construction: Gateway cloning was performed using methods and reagents from the Invitrogen Gateway cloning system (Invitrogen, USA). The cloned full-length wild type melon PH gene was used as a template for a PCR via primers listed in Supplementary Table 2 . The cloned PCR product was delivered via standard protocol into the yeast expression destination vector pYES-DEST52, resulting in pYES-DEST52- CmPH . In a similar fashion, the mutant (‘Dulce’) melon PH gene was cloned to obtain pYES-DEST52- CmPH’Dulce’. Stable Agrobacterium -mediated plant transformation Agrobacterium -mediated plant transformation was performed as described in Supplementary Methods . Transient expression Preparation of Agrobacterium for transient expression: Preparation of the Agrobacterium infiltration medium for transient expression was executed as described previously [44] . Transient expression in melon: In full-size, non-ripe ( ca 30 days past pollination) melon fruits (non-sour NILs described above), 1 ml of the described YFP or GFP SlPH Agrobacterium infiltration medium was injected via a 20G 0.8 × 40 mm needle ~20 mm deep into the fleshy mesocarp at the equatorial portion, as modified from the technique used for tomato fruit [45] . The fruit was imaged 10 days after injection. Transient expression in tobacco: Transient expression of HDEL-RFP (via the described transformed Agrobacterium ) was performed in leaves, stem and ovary of stably transformed YFP - SlPH tobacco, modified from the technique used for tomato leaves [46] and capsules, as modified from the technique used for tomato fruit [45] . The described infiltration medium was introduced into various plant organs as follows: In young tobacco leaves, 1 ml of the medium was injected via a needleless 5 ml syringe into the abaxial side. In 20 mm green tobacco fruit, the medium was injected via a 20G 0.8 × 40 mm needle half way into the fleshy mesocarp along the capsule’s polar axis until drops were seen exuding from the surrounding petals. All of the tissues described above were imaged 48 h after injection. Protoplast and vacuole preparation Protoplast isolation: Leaf mesophyll protoplasts were isolated from YFP - SlPH transformed tobacco. Protoplasts from YFP - SlPH transformed tobacco plants were produced according to the procedure described by Draper et al . [37] and incubated in the dark for 48 h at 27 °C before imaging. Vacuole partial lysis: Partial lysis of tobacco protoplasts was adapted from the protocol used in grape protoplasts [46] . The protoplast suspension was added to 2.5 volumes of the prewarmed lysis buffer (42 °C), a solution with reduced osmotic strength containing 0.2 M mannitol, 10% Ficoll (w/v), 15 mM EDTA, 10 mM MOPS, pH 8.0, resulting in the release of intact vacuoles. Visualization of live vacuoles was performed via an addition of 100 mM Neutral Red dye (#N4638 Sigma-Aldrich; http://www.sigmaaldrich.com ) in 80 mM phosphate buffer pH 7.2. Microscopy and cellular localization Microscopy methods presented in Supplementary Methods . Uptake of nucleosides and organic acids in yeast cells Measuring the uptake of radioactive nucleosides and organic acids in yeast cells is based on the methods described previously by Möhlmann et al . [47] with the following changes. SC medium for induction of PH gene contained the amino acids Leu, Lys, His, Met and 2% Raffinose as a carbon source, as well as 1% galactose. The yeast expression vectors used were pYES (empty), pYES-DEST52- CmPH and pYES-DEST52- CmPHmut and the Saccharomyces cerevisiae strain BY4743. Chromatography The nucleosides were identified by high performance LC–MS and their levels were measured using HPLC-DAD method (see Supplementary Methods ). The untargeted metabolite analysis was carried using high performance LC–MS and gas chromatography–mass spectrometry methods (see Supplementary Methods ). Protein transmembrane domain modelling Transmembrane prediction was performed as described in Supplementary Methods . PH gene expression analysis Total RNA was extracted from the flesh tissue of five pooled mature fruits of each of RI lines, representing the 11 highest and 13 lowest pH values. Strand-specific RNA-seq libraries were constructed from the total RNA as described previously [48] and sequenced on the Illumina HiSeq platform. RNA-Seq reads were first aligned to ribosomal RNA sequences using Bowtie [49] to remove possible rRNA contaminations. The resulting filtered reads were aligned to the melon genome [17] using TopHat [50] . Following alignments, raw counts for the PH gene were obtained and normalized to reads per kilobase of exon model per million mapped reads. Yeast growth conditions and transformation Selective liquid media for uracil auxothrophic growth, −URA+sugar, contained 0.5% ammonium sulphate (A901217 Merck, Germany), 0.17% yeast nitrogen base without amino acids (Y0626 Sigma, USA), 0.2% Bacto casamino acids (223050 BD, USA), 0.004% adenine (A-9126 Sigma, Germany), 0.008% tryptophan (T-0254 Sigma, USA) and 110 mM of either galactose (G0625 Sigma-Aldrich, Italy) or glucose (G0802 Duchefa Biochemie, The Netherlands). All yeast cells were incubated at 30 °C with shaking (150 g ) with an air:culture ratio greater than 5:1. Transformation of yeast vectors, pYES-DEST52 or pESC-URA, was performed on the Saccharomyces cerevisiae strain BY4743 (MATa/α his3Δ1/his3Δ1 leu2Δ0/leu2Δ0 LYS2/lys2Δ0 met15Δ0/MET15 ura3Δ0/ura3Δ0) (EUROSCARF, Germany) using standard protocol [51] . Nucleoside feeding test pYES-DEST52 and pYES-DEST52- CmpH yeast transformed cells were grown in 600 ml selective liquid media (glucose) to a stationary phase for 24 h to an O.D. (optical density) of 3.75. The cells were pelleted at 5,000 g , washed with 40 ml water and resuspended in galactose selective liquid media containing 13 mM adenosine to the same O.D. The cells were pelleted immediately and after 4 h of incubation at 30 °C with shaking (150 g ), washed twice with 20 ml sterile DDW and frozen in liquid nitrogen. Nucleoside extraction The frozen yeast pellet (~200 μl) was resuspended in 1 ml of methanol:water (1:1, v-v), vortexed for 2 min, sonicated for 30 min, vortexed for 2 min again and centrifuged at 15,000 g . The liquid phase was filtered using 0.2 μm PTFE membrane filters and transferred into HPLC vials for further analysis in HPLC-DAD. Phylogenetic analysis The protein sequences were aligned using Muscle algorithm and the phylogenetic tree was analysed and visualized by the SeaView v4.3.5 programme using the maximum likelihood method by PhyML 3.0 (ref. 52 ) with the following settings: model—LG; the approximate likelihood ratio test Shimodaira–Hasegawa-like procedure was used as a statistical test to calculate branch support—approximate likelihood ratio test (Shimodaira–Hasegawa-like); invariable sites—optimized; across site rate variation—optimized; tree searching operations—best for NNI and SPR; starting tree—BioNJ, optimize tree topology. The numbers on the branches indicate the fraction of bootstrap iterations supporting each node. The accession numbers of the proteins used for the preparation of this tree and the organism names are listed in Supplementary Table 3 . How to cite this article : Cohen, S. et al . The PH gene determines fruit acidity and contributed to the evolution of sweet melons. Nat. Commun. 5:4026 doi: 10.1038/ncomms5026 (2014).